Size limits the formation of liquid jets during bubble bursting A bubble reaching an air–liquid interface usually bursts and forms a liquid jet. Jetting is relevant to climate and health as it is a source of aerosol droplets from breaking waves. Jetting has been observed for large bubbles with radii of R ≫ 100 μm. However, few studies have been devoted to small bubbles ( R <100 μm) despite the entrainment of a large number of such bubbles in sea water. Here we show that jet formation is inhibited by bubble size; a jet is not formed during bursting for bubbles smaller than a critical size. Using ultrafast X-ray and optical imaging methods, we build a phase diagram for jetting and the absence of jetting. Our results demonstrate that jetting in bubble bursting is analogous to pinching-off in liquid coalescence. The coalescence mechanism for bubble bursting may be useful in preventing jet formation in industry and improving climate models concerning aerosol production. The bursting of bubbles is an important transport mechanism in physical, chemical and biological processes occurring at the air–liquid interface [1] , [2] , [3] , [4] , [5] , [6] , [7] , [8] , [9] , [10] , [11] , [12] , [13] , [14] , [15] , [16] , [17] , [18] . Aerosol production from bursting bubbles is commonly used for enlivenment by releasing aromatic aerosols from sparkling drinks [8] , [9] . Most marine aerosols are formed through the bursting process of bubbles entrained by breaking waves [10] , [11] , [12] , [13] . They have been studied experimentally [14] , [15] and numerically [16] , [17] for over half a century [1] , [2] , [3] because of their great significance in cloud and hurricane dynamics, the Earth's radiative balance and biogeochemical cycles [10] , [11] . A tremendous number of bubbles with radii ( R ) smaller than 100 μm are entrained into sea water [10] . According to previous observations, bursting of large bubbles ( R ≫ 100 μm) exhibits the formation of jets and aerosols [1] , [2] , [12] . For small bubbles ( R <100 μm), however, jet formation has not been experimentally investigated despite the expected absence of jetting behaviour [12] , [13] . The visualization of bursting in bubbles of such sizes is a challenge because they rise extremely slowly and their bursting events become sparse at calm liquid surfaces [13] , [18] .Here we present direct visualization of bubble bursting using ultrafast X-ray and optical imaging in a drop-impact situation. High-resolution and high-penetration X-ray imaging enables us to precisely track the surface evolution of small bubbles, which is essential to elucidate the mechanism of jetting in bubble bursting. Optical imaging for bubble bursting A drop-impact setup is used to facilitate the bursting event and to control the bubble size ( R <100 μm). When a drop impacts on a solid substrate, a small amount of air is rapidly trapped and contracted into a spherical bubble [19] , [20] , [21] . The air entrainment between the liquid free surface and the substrate is a robust phenomenon, regardless of the liquid or the substrate [21] . The entrapped bubble, as it rises up and reaches the free surface, eventually bursts [21] . The bursting process is not significantly affected by the substrate for such small bubbles whether the substrate is very close to, touches or very far from the bubbles, as seen by high sphericities of bubbles. Of course, the presence of the substrate beneath the bubbles may affect the jetting velocity by changing the motion of the capillary waves [22] . We note that the dynamic fluctuation of the free surface (with a depth of 70–300 μm) after impact significantly increases the chance for the bubble to contact the free surface. The bubble size is easily controlled by changing the falling height or the drop size [20] . The bursting events were first visualized with varying bubble sizes using ultrafast optical microscopy ( Fig. 1 ), showing jetting at R ∼ 35 μm ( Supplementary Movie 1 ) and the absence of jetting at R ∼ 20 μm ( Supplementary Movie 2 ) in ethanol ( Fig. 1a ); jetting at R ∼ 50 μm ( Supplementary Movie 3 ) and the absence of jetting at R ∼ 43 μm ( Supplementary Movie 4 ) in decalin ( Fig. 1b ). Here we find that jet formation, as demonstrated by the emission of aerosol droplets into the atmosphere, occurs only for the bubbles larger than a critical size. The size threshold for jetting is dependent on the liquid properties; for instance, the threshold is smaller in ethanol than in decalin. For generality, we tested five low-viscosity liquids (dynamic viscosities of ∼ 1 cP): water, ethanol, dodecane, tridecane and decalin. The size limitation in jetting was observed for all small bubbles ( R <100 μm), for all of the liquids except water. This finding implies that jet formation is not necessarily induced by bursting and is limited by bubble size. 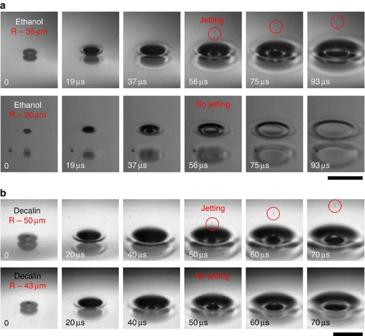Figure 1: Size limitation of jetting from bursting bubbles. Bubble bursting from small bubbles (R<100 μm) in a typical drop-impact experiment. A liquid drop that freely falls from a height onto a solid surface robustly forms a single small bubble after impact. Once a trapped bubble reaches the fluctuated liquid free surface, it rapidly bursts. The critical size differs with the liquid. (a) Ultrafast optical images of jetting (upper, the bubble radiusR∼35 μm) and the absence of jetting (lower,R∼20 μm) in ethanol. Scale bar, 200 μm. (b) Another example of jetting (upper,R∼50 μm) and the absence of jetting (lower,R∼43 μm) in decalin. Scale bar, 150 μm. The jet formation is characterized by the emission of aerosol droplets into the atmosphere (marked as circles). Dodecane and tridecane show a similar size limitation for jetting, but water always shows jetting. Figure 1: Size limitation of jetting from bursting bubbles. Bubble bursting from small bubbles ( R <100 μm) in a typical drop-impact experiment. A liquid drop that freely falls from a height onto a solid surface robustly forms a single small bubble after impact. Once a trapped bubble reaches the fluctuated liquid free surface, it rapidly bursts. The critical size differs with the liquid. ( a ) Ultrafast optical images of jetting (upper, the bubble radius R ∼ 35 μm) and the absence of jetting (lower, R ∼ 20 μm) in ethanol. Scale bar, 200 μm. ( b ) Another example of jetting (upper, R ∼ 50 μm) and the absence of jetting (lower, R ∼ 43 μm) in decalin. Scale bar, 150 μm. The jet formation is characterized by the emission of aerosol droplets into the atmosphere (marked as circles). Dodecane and tridecane show a similar size limitation for jetting, but water always shows jetting. Full size image X-ray imaging for bubble bursting It is a critical challenge to clearly track the surface evolution of small bubbles ( R <100 μm) beneath liquid with ultrafast optical imaging; the time resolution is adequate (μs), but the spatial resolution in liquid is insufficient mainly due to the strong reflection or scattering effects that are usually associated with visible light imaging [23] . To resolve this problem, we adopted ultrafast X-ray phase-contrast imaging, which combines X-ray phase-contrast microscopy with an ultrafast camera [23] , [24] . The precise tracking of the liquid–air interface was made possible because of the high penetration capability of X-ray photons [25] , [26] , [27] , enabling us to clearly observe the bursting process for small bubbles ( R <100 μm), for instance, in water ( R =26.5 μm, Fig. 2a ; Supplementary Movie 5 ) and in ethanol ( R =24.5 μm, Fig. 2b ; Supplementary Movie 6 ). Specifically, X-ray imaging technique allows us to visualize the surface shape of small bubbles, which is essential to elucidate the mechanism of jetting in bubble bursting. 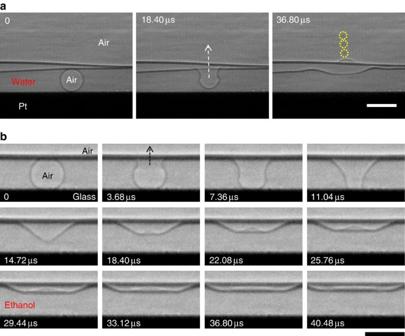Figure 2: Bubble bursting of small bubbles. X-ray phase-contrast imaging was adopted to clearly reveal the surface evolution of bubbles (20 μm<R<100 μm) beneath liquid using the high penetration capability of X-ray photons. The constant falling height (35 mm) in the drop-impact experiments generated bubbles with the same volume, regardless of the liquid or substrate. (a) Ultrafast X-ray imaging of a bursting bubble (R=26.5 μm) in water on a platinum substrate. The images demonstrate the jet formation from a bubble. The radii of the daughter aerosol droplets were 2–4 μm (marked as circles), 15% of the parent bubble size, consistent with the previous observation (ref.3). Scale bar, 60 μm. (b) Ultrafast X-ray imaging of a bursting bubble (R=24.5 μm) in ethanol on a glass substrate. The images show no jetting for such a small bubble. Scale bar, 60 μm. Figure 2: Bubble bursting of small bubbles. X-ray phase-contrast imaging was adopted to clearly reveal the surface evolution of bubbles (20 μm< R <100 μm) beneath liquid using the high penetration capability of X-ray photons. The constant falling height (35 mm) in the drop-impact experiments generated bubbles with the same volume, regardless of the liquid or substrate. ( a ) Ultrafast X-ray imaging of a bursting bubble ( R =26.5 μm) in water on a platinum substrate. The images demonstrate the jet formation from a bubble. The radii of the daughter aerosol droplets were 2–4 μm (marked as circles), 15% of the parent bubble size, consistent with the previous observation (ref. 3 ). Scale bar, 60 μm. ( b ) Ultrafast X-ray imaging of a bursting bubble ( R =24.5 μm) in ethanol on a glass substrate. The images show no jetting for such a small bubble. Scale bar, 60 μm. Full size image The most important feature in the initial bursting process is a significant deformation of the bubble shape for small bubbles ( R <100 μm). Before the bursting event (when t <0), the equilibrium shape of the bubble is spherical because of its small size ( R ≪ the capillary length, for example, ∼ 2.7 mm for water). At the rupture initiation ( t =0), the liquid film between the bubble and the atmosphere retracts very rapidly; the retraction speed is ∼ 10 m s −1 for typical low-viscosity liquid films as thick as 1 μm [11] , [15] . This rapid retraction results in an instantaneous deformation of the bubble shape, similar to a cone shape (see the bubble shape at 14.72 μs in Fig. 2b ). The quantitative measurement of the shape deformation by ultrafast X-ray imaging is an essential clue to elucidating the jet-formation mechanism discussed below. Critical condition for jetting In general, jet formation occurs through the convergence of capillary waves along the liquid–air interface [13] , [14] , [16] . For capillary waves with a wavelength much smaller than the bubble radius ( R ), the wave velocity is ν w =( σk / ρ ) 1/2 where k is the wavenumber, σ is the surface tension and ρ is the density [28] , [29] . The travelling distance of waves to reach the bottom apex is measured as L ∼ 0.5 πR ( Fig. 3 ) for small bubbles ( R ∼ 25 μm), and therefore, the travelling time of the waves is t ∼ 0.5 πR /( σk / ρ ) 1/2 . The damping rate of the waves, associated with the viscous dissipation, is D =2 μ k 2 / ρ , where μ is the liquid dynamic viscosity [28] . A condition for a significant amount of momentum to reach the bottom apex is given as Dt <1 (ref. 28 ). Equivalently, this condition is π ( Rk ) 3/2 Oh <1. Here the Ohnesorge number, Oh=μ/( ρσR ) 1/2 , is a non-dimensionalized viscosity that is the ratio of typical viscous and surface forces [28] . This relationship suggests the existence of a critical Ohnesorge number (Oh*), above which jetting does not occur because viscous stresses suppress jetting by dissipating capillary waves. 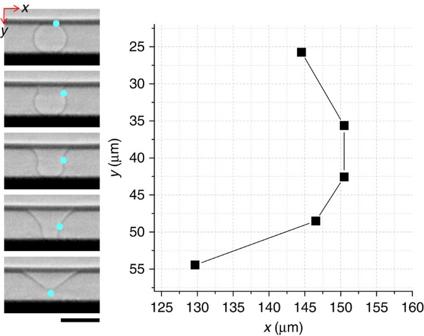Figure 3: Travel in capillary waves. In a single bursting event, the travelling distance of capillary waves was graphically measured asL∼0.53πR, whereRis the initial bubble radius, from the snapshots (Fig. 2b) obtained by ultrafast X-ray imaging. The blue dot indicates the wave crest. The average value from five different events isL∼0.53±0.02πR, and the approximationL≈0.5πRwas used as the travelling distance in the text. Scale bar, 60 μm. Figure 3: Travel in capillary waves. In a single bursting event, the travelling distance of capillary waves was graphically measured as L ∼ 0.53 πR , where R is the initial bubble radius, from the snapshots ( Fig. 2b ) obtained by ultrafast X-ray imaging. The blue dot indicates the wave crest. The average value from five different events is L ∼ 0.53±0.02 πR , and the approximation L ≈0.5 πR was used as the travelling distance in the text. Scale bar, 60 μm. Full size image Jetting and pinching off The above argument for bubble bursting is similar to that for liquid coalescence [28] except for the significant deformation in bubble bursting. The two processes can be understood as a coalescence of two parent clusters, namely, the coalescence of a bubble into the atmosphere (reservoir) and of a liquid drop into a flat liquid reservoir. For liquid coalescence, there is a hydrodynamic singularity, known as 'pinching-off' or satellite drop formation, which is associated with the ability of capillary waves to stretch the drop surface and deliver momentum on the drop summit [28] . One way that jetting differs from pinching-off is its significant reduction in the travelling distance; L is reduced to ≈0.5 πR for bursting whereas L ≈ πR for liquid coalescence [28] . Oh* for a droplet on a flat liquid surface was measured as ≈0.026 at very low Bond numbers (<0.01) (Bo= ρgR 2 / σ (a non-dimensional weight that compares gravitational and surface forces)) [28] . With almost half of the travelling distance ( L ≈0.5 πR ), we can predict Oh*≈0.052 in jetting for small bubbles (Bo<0.001). It is conceivable that the decrease in the travelling distance leads to a reduction of the travelling time and thus an increase in the critical Ohnesorge number. Size limitation The size threshold for jetting is crucial to understanding the bubble-mediated jetting process. The critical Ohnesorge number immediately determines the minimum bubble radius, R *= μ 2 /[ ρσ (Oh*) 2 ], below which jetting does not occur. For a given liquid (at fixed values of μ, ρ and σ ), R * is estimated from Oh*≈0.052 as ≈4, 26, 34, 48 and 54 μm for water, ethanol, dodecane, decalin and tridecane, respectively. The direct visualization of the bubbles ( R =26.5 μm) in water and in ethanol ( R =24.5 μm) supports our estimation of R *: jetting occurs in water for R > R * ( Fig. 2a ), whereas no jetting occurs in ethanol for R < R * ( Fig. 2b ). The coalescence mechanism for bubble bursting suggests the existence of a bifurcation of jetting and no jetting depending on the bubble size, particularly for small bubbles ( R <100 μm). Phase diagram To test the coalescence mechanism for bubble bursting, a wide range of bubble size (20 μm< R <300 μm) was investigated for ethanol, dodecane, tridecane and decalin using ultrafast optical imaging. Bubbles with R >100 μm were taken by a direct injection into thick liquids, while those with R <100 μm were taken by a drop-impact setup. A phase diagram for jetting and the absence of jetting was obtained in terms of the Oh (to describe the capillarity effects) and the Bo numbers (to describe the gravity effects) ( Fig. 4a ). In this diagram, the critical Ohnesorge number is found to be Oh*≈0.052±0.005, which is consistent with our prediction based on the coalescence mechanism for small bubbles (Bo<10 −3 ). The critical bubble sizes ( R *), estimated from Oh*≈0.052, are well matched with the experimental data for the tested liquids. For water, we also investigated bubble bursting with the only observation of jetting in all bubbles tested (20 μm< R <300 μm), consistent with the estimate of R *≈4 μm. 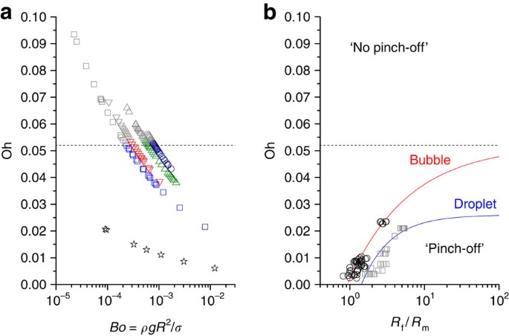Figure 4: Phase diagram for jet formation from bursting bubbles. (a) Experimental results for a wide range (20 μm<R<300 μm) of bubble sizes in water (star), ethanol (square), dodecane (downward triangle), decalin (upward triangle) and tridecane (circle) plotted in a phase diagram in terms of the Ohnesorge (Oh, for the capillarity effects) and Bond numbers (Bo, for the buoyancy effects). The zone of Oh<Oh* describes jetting cases, whereas the zone of Oh>Oh* indicates the absence of jetting. The critical Ohnesorge number is marked at Oh*≈0.052±0.005 (marked by the dashed line) for negligible buoyancy effects (at Bo<10−3). (b) General coalescence phase diagram in terms of the parent size ratio,Rf/Rm(Rf>Rm). Typical droplet–droplet (squares, ref.30) and bubble–bubble (circles, ref.31) systems show similar size ratio dependences of Oh*, below which pinching-off (or jetting) occurs. The droplet coalescence reaches the asymptote of Oh∞*=0.026 (ref.28) forRf=∞ or a droplet on a flat liquid surface. The asymptote for bubble is suggested to be around Oh∞*=0.052 (dashed line). The parent size ratio dependences of Oh* are fitted by an asymptotic function of Oh*=Oh∞*−a(Rf/Rm)−bwith Oh∞*=0.052 (this paper),a=0.050, andb=0.535 for bubble and with Oh∞*=0.026 (ref.28),a=0.039, andb=1.128 for droplet (solid lines). Figure 4: Phase diagram for jet formation from bursting bubbles. ( a ) Experimental results for a wide range (20 μm< R <300 μm) of bubble sizes in water (star), ethanol (square), dodecane (downward triangle), decalin (upward triangle) and tridecane (circle) plotted in a phase diagram in terms of the Ohnesorge (Oh, for the capillarity effects) and Bond numbers (Bo, for the buoyancy effects). The zone of Oh<Oh* describes jetting cases, whereas the zone of Oh>Oh* indicates the absence of jetting. The critical Ohnesorge number is marked at Oh*≈0.052±0.005 (marked by the dashed line) for negligible buoyancy effects (at Bo<10 −3 ). ( b ) General coalescence phase diagram in terms of the parent size ratio, R f / R m ( R f > R m ). Typical droplet–droplet (squares, ref. 30 ) and bubble–bubble (circles, ref. 31 ) systems show similar size ratio dependences of Oh*, below which pinching-off (or jetting) occurs. The droplet coalescence reaches the asymptote of Oh ∞ *=0.026 (ref. 28 ) for R f =∞ or a droplet on a flat liquid surface. The asymptote for bubble is suggested to be around Oh ∞ *=0.052 (dashed line). The parent size ratio dependences of Oh* are fitted by an asymptotic function of Oh*=Oh ∞ *− a ( R f / R m ) − b with Oh ∞ *=0.052 (this paper), a =0.050, and b =0.535 for bubble and with Oh ∞ *=0.026 (ref. 28 ), a =0.039, and b =1.128 for droplet (solid lines). Full size image To gain insight into the mechanism behind bubble bursting, we compare bursting case with the other coalescence cases. Coalescence processes have been well studied for droplet–droplet or bubble–bubble cases: the critical Oh number for the ejection of daughter droplets (or bubbles) from parent droplets (or bubbles) increases with the size ratio, R f / R m ( R f > R m : f=father and m=mother) [30] , [31] , as illustrated in Figure 4b . For drop–drop case, the critical Oh number reaches the asymptote (Oh ∞ *) of 0.026 (refs 28 , 29 ) at the limit case of R f =∞, that is, a droplet on a flat liquid surface [28] , [29] . However, the asymptote at R f =∞ for bubble (that is, a bubble beneath a flat liquid surface) has not been established yet. Daughter aerosols are ejected in bubble bursting, whereas daughter bubbles are generated in bubble–bubble coalescence. The critical Oh number for bubble bursting is around 0.052 ( Fig. 4a ). The parent size ratio dependences of Oh* ( Fig. 4b ) can be described as a typical asymptotic function of Oh*=Oh ∞ *− a ( R f / R m ) − b ( a and b >0). By fitting the overall data [28] , [29] , [30] , [31] with Oh ∞ *=0.052 (this paper), a =0.050, and b =0.535 for bubble, and with Oh ∞ *=0.026 (ref. 28 ), a =0.039, and b =1.128 for droplet, we obtain a general coalescence phase diagram for droplet and bubble in terms of the parent size ratio ( Fig. 4b ). The size ratio dependences of Oh* are attributed to the pressure difference between two parents, [30] . In this phase diagram, the cases of no jetting at Oh ≪ Oh* for large bubbles ( R >several mm) (ref. 17 ) are excluded. This diagram implies that jetting in bubble and pinching-off in droplet are identical singularities associated with capillary waves and can be identified by the critical Oh values. The critical discrepancy between bubble and droplet is the magnitude of Oh*: Oh* is almost twice for bubble than for droplet. This is attributed to the shortened travelling length of capillary waves for bubble. What drives the reduction of the travelling length? Here we show two intrinsic features of bubble bursting: (i) the significant surface deformation driven by the rapid rupture and (ii) the partial gas ejection enhanced by the large pressure difference. These features offer the physical bases of the reduced travelling length for bubble and thus the increased critical Oh value. The rupture dynamics of low-viscosity liquid films has a scaling of r ∼ ( σR / ρ ) 1/4 t 1/2 where r is the neck radius by balancing inertia against surface tension [23] , [32] , [33] . The t 1/2 dependence is indeed observed in ethanol and in decalin ( Fig. 5a ) regardless of jet formation, indicating the inertial rupture dynamics [11] , [34] . The prefactor is 12.5±1.5 from r [μm] versus t 1/2 [μs 1/2 ] ( Fig. 5a ). Even in the rescaling of the rupture dynamics with r / R and t / τ where τ =( ρR 3 / σ ) 1/2 , the prefactors, that is, the slopes become different for each liquid [33] , for instance, as 2.5 for ethanol and 2.0 for decalin ( Fig. 5b ). The retraction speed, obtained by the differentiation of r with regard to t , U =d r /d t >6 m s −1 for t <1 μs. This estimate well agrees with the typical inertial rupture speed, U =(2 σ / ρh ) 1/2 , which is generally of order 10 m s −1 (the thickness, h ∼ 1 μm) [15] , [34] . This agreement also suggests that the retraction dynamics is driven by the rapid inertial rupture. We note that the rapid rupture for bubble intrinsically leads to the significant surface deformation at rupture, as clearly demonstrated in Figure 2 . 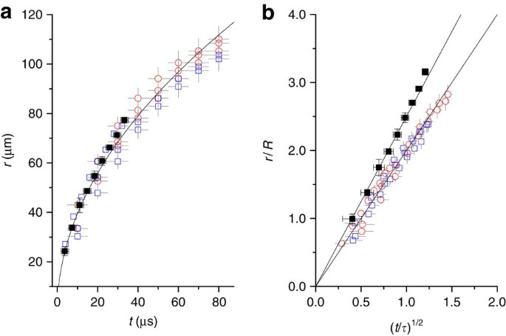Figure 5: Rapid rupture dynamics for bubbles. (a) The growth of the neck radius (r) with time (t) for ethanol (no jetting case) and for decalin (jetting and no jetting cases). The neck growth has a scaling ofr∼(σR/ρ)1/4t1/2for low-viscosity liquids. Thet1/2dependences observed in ethanol and in decalin, regardless of jet formation, indicate the inertial rupture dynamics. The average data for ethanol from three events (solid squares,R∼25 μm, Oh>Oh*) were taken by X-ray imaging, and the data of individual events for decalin from no jetting (open squares,R=36.69, 37.48 and 43.07 μm, Oh>Oh*) and jetting (open circles,R=49.4, 45.46 and 46.26 μm, Oh<Oh*) cases were taken by optical imaging. The prefactor is fitted as 12.5±1.5 fromr[μm] versust1/2[μs1/2]. (b) The normalized neck growth dynamics by rescalingr/Randt/τwhereτ=(ρR3/σ)1/2shows the different prefactors of 2.5 for ethanol and 2.0 for decalin. The linearity again supports the inertial rupture dynamics. Error bars come from a standard deviation derived from measurement errors (errors: ± 5% ofrand ± Δtof minimum interval). Figure 5: Rapid rupture dynamics for bubbles. ( a ) The growth of the neck radius ( r ) with time ( t ) for ethanol (no jetting case) and for decalin (jetting and no jetting cases). The neck growth has a scaling of r ∼ ( σR / ρ ) 1/4 t 1/2 for low-viscosity liquids. The t 1/2 dependences observed in ethanol and in decalin, regardless of jet formation, indicate the inertial rupture dynamics. The average data for ethanol from three events (solid squares, R ∼ 25 μm, Oh>Oh*) were taken by X-ray imaging, and the data of individual events for decalin from no jetting (open squares, R =36.69, 37.48 and 43.07 μm, Oh>Oh*) and jetting (open circles, R =49.4, 45.46 and 46.26 μm, Oh<Oh*) cases were taken by optical imaging. The prefactor is fitted as 12.5±1.5 from r [μm] versus t 1/2 [μs 1/2 ]. ( b ) The normalized neck growth dynamics by rescaling r / R and t / τ where τ =( ρR 3 / σ ) 1/2 shows the different prefactors of 2.5 for ethanol and 2.0 for decalin. The linearity again supports the inertial rupture dynamics. Error bars come from a standard deviation derived from measurement errors (errors: ± 5% of r and ± Δ t of minimum interval). Full size image The rapid rupture dynamics deforms a spherical bubble to a cone shape prior to jet formation, as usually observed [1] , [2] , [7] , [14] , [16] , [31] . The cone shape implies a significant partial gas ejection from the deformed bubble into the atmosphere, causing a large volume shrinkage, Δ V = V 0 − V g where V 0 is the initial gas volume and V g is the gas volume at jet formation. The partial gas ejection can be significantly enhanced as the pressure difference, Δ p =2 σ / R , increases. 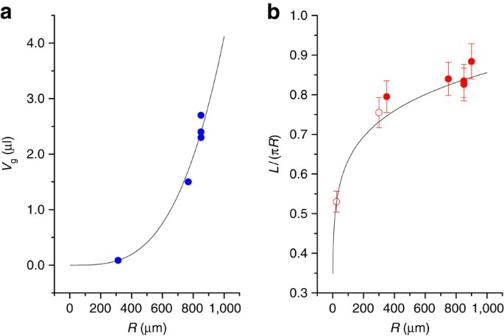Figure 6: Partial gas ejection for bubbles. (a) The gas volume at jet formation (Vg) versus the initial radius (R) plot, measured from literature (refs1,2,7,14,16; solid circles), fitted by a power law,Vg/V0∼RcwhereV0is the initial gas volume (the solid line:Vg=9.75V0R0.33). The partial gas ejection is enhanced as the pressure difference Δp=2σ/Rincreases. (b) The bubble size dependence of the travelling length (L) normalized by the original travelling length (πR), measured from literature (refs1,7,14,16,31; solid circles) and ours (open circles), fitted byL/πR∼Rd(the solid line:L/πR=2.1R0.13). The exponent ofd=0.13 is well matched toc/3=0.11, assuming (L/πR) is proportional to (Vg/V0)1/3. Error bars, 5% measurement errors. From literature for bubble bursting [1] , [2] , [7] , [14] , [16] , the gas volume ( V g ) versus the initial radius ( R ) is plotted in Figure 6a and can be fitted by a power law, V g / V 0 ∼ R c (the solid line: V g =9.75 V 0 R 0.33 ). The bubble-size dependence of the travelling length ( L ) normalized by the original travelling length ( πR ), measured from literature [1] , [7] , [14] , [16] , [31] , is plotted in Figure 6b and can be fitted by L / πR ∼ R d (the solid line: L / πR =2.1 R 0.13 ). The exponent of d =0.13 is well matched to c /3=0.11, assuming that ( L / πR ) is proportional to ( V g / V 0 ) 1/3 . This finding also suggests that the partial gas rejection in bubble bursting leads to the reduction in the travelling length and therefore induces the increase in the critical Oh number. Figure 6: Partial gas ejection for bubbles. ( a ) The gas volume at jet formation ( V g ) versus the initial radius ( R ) plot, measured from literature (refs 1 , 2 , 7 , 14 , 16 ; solid circles), fitted by a power law, V g / V 0 ∼ R c where V 0 is the initial gas volume (the solid line: V g =9.75 V 0 R 0.33 ). The partial gas ejection is enhanced as the pressure difference Δ p =2 σ / R increases. ( b ) The bubble size dependence of the travelling length ( L ) normalized by the original travelling length ( πR ), measured from literature (refs 1 , 7 , 14 , 16 , 31 ; solid circles) and ours (open circles), fitted by L / πR ∼ R d (the solid line: L / πR =2.1 R 0.13 ). The exponent of d =0.13 is well matched to c /3=0.11, assuming ( L / πR ) is proportional to ( V g / V 0 ) 1/3 . Error bars, 5% measurement errors. Full size image Bubble bursting, as a key liquid-to-air transfer process, is important in atmospheric aerosol production and the scavenging activity of biological materials, for physical oceanography, atmospheric chemistry, weather and climate modelling, chemical engineering and human health. For instance, dinoflagellate cell collection and lysis can be driven by bursting processes in the surf zone. The subsequent aerosolization of neurotoxins in the cell cytoplasm may cause a respiratory hazard. The size limitation of jetting from bursting bubbles in low-viscosity liquids has been verified for the first time thanks to direct visualization with ultrafast X-ray phase-contrast imaging for bubbles with small radii ( R <100 μm). The jetting process of bursting bubbles is associated with the convergence of capillary waves, described by the critical Ohnesorge number, similar to the coalescence mechanism of liquid drops. The analogy between jetting and pinching-off enables us to understand bubble bursting as gas coalescence. This finding will be useful in controlling the bursting process in refreshing drinks [9] by changing the surface tension, viscosity or density, namely, by adding surfactants or functional ingredients. In particular, the size threshold for aerosol production is expected to increase with high viscosity, low surface tension or low density. The increase of the size threshold is desirable in industrial situations such as glass manufacturing or biotechnology [11] to prevent jetting. The size threshold for the emission of aerosol droplets from bursting bubbles in the ocean to the atmosphere is significant for understanding the size distribution of aerosols in climate scenarios. Materials We tested typical low-viscosity liquids: pure water (Millipore), ethanol (Merck, ≥99%), dodecane (Sigma-Aldrich, ReagentPlus, ≥99%), tridecane (Sigma-Aldrich, ≥99%) and decalin (Sigma-Aldrich, mixture of cis and trans, anhydrous, ≥99%). Their properties were obtained from the literature [35] , [36] , [37] , [38] , [39] , [40] , [41] , [42] , [43] and used to estimate the minimum bubble radius for jet formation, R *= μ 2 /[ ρσ (Oh*) 2 ], based on Oh*=0.052 ( Table 1 ). Platinum and glass were used as flat solid substrates. Table 1 Liquid properties and size thresholds. Full size table X-ray imaging The high spatial and temporal resolutions required for the observation of bubble bursting were achieved by an intense white (full energy spectrum) X-ray beam with a peak irradiance of ∼ 10 14 ph s −1 mm −2 per 0.1% b.w. delivered by the XOR 32-ID undulator beamline of the Advanced Photon Source of the Argonne National Laboratory [23] . Using this specific synchrotron beamline, we were able to achieve direct visualization of ultrafast bursting dynamics on the μs timescale. In particular, we took images with a 472 ns exposure time and interframe time (a multiple of the storage ring period of ∼ 3.68 μs) using an ultrafast camera (Photron Fastcam SA 1.1). The camera was synchronized and gated to the X-ray pulses. Any possible X-ray-induced changes in the liquid properties are negligible in these very short irradiation times [26] , [27] . A laser beam was used to sense the falling drop (2 μl) from a constant height of 35 mm and to trigger the camera to take images [23] . Phase diagram To obtain the phase diagram using ultrafast optical microscopy in drop-impact experiments, the bubble size was controlled by changing the falling height and/or the drop size. The spatial resolutions of the two imaging methods were sufficient to identify the absence of jetting because the aerosol sizes, which are 15% of the mother bubble sizes [3] , are larger than 1 μm except for water at the critical bubble sizes. How to cite this article: Lee, J. S. et al . Size limits the formation of liquid jets during bubble bursting. Nat. Commun. 2:367 doi: 10.1038/ncomms1369 (2011).